A downy mildew effector evades recognition by polymorphism of expression and subcellular localization Pathogen co-evolution with plants involves selection for evasion of host surveillance systems. The oomycete Hyaloperonospora arabidopsidis ( Hpa ) causes downy mildew on Arabidopsis, and race-specific interactions between Arabidopsis accessions and Hpa isolates fit the gene-for-gene model in which host resistance or susceptibility are determined by matching pairs of plant Resistance ( R ) genes and pathogen Avirulence ( AVR ) genes. Arabidopsis Col-0 carries R gene RPP4 that confers resistance to Hpa isolates Emoy2 and Emwa1, but its cognate recognized effector(s) were unknown. We report here the identification of the Emoy2 AVR effector gene recognized by RPP4 and show resistance-breaking isolates of Hpa on RPP4 -containing Arabidopsis carry the alleles that either are not expressed, or show cytoplasmic instead of nuclear subcellular localization. Plants and pathogens have co-evolved in a defensive and offensive battle for survival. Pathogens promote infection success by secreting effector proteins that modulate a variety of plant cellular functions, thus rendering hosts more susceptible. In turn, plants have evolved intracellular receptors containing nucleotide-binding and leucine-rich repeat domains (NLRs), that can directly or indirectly detect pathogen effectors. Disease Resistance (R) genes usually encode NLR proteins, and extensive genetic variation is observed at NLR-encoding loci. Recognized effectors are encoded by so-called Avirulence ( AVR ) genes and recognition by R proteins leads to effector-triggered immunity (ETI), often culminating in a hypersensitive response (HR) cell death [1] . Allelic variation, including loss-of-function mutations, in an AVR gene can enable a pathogen race to evade recognition and cause disease on plants that carry the cognate R gene. Arabidopsis is a host for the biotrophic oomycete Hyaloperonospora arabidopsidis ( Hpa ; formerly Peronospora parasitica or Hyaloperonospora parasitica ), a downy mildew pathogen. This model pathosystem has revealed cognate host R and pathogen AVR genes, termed RPP (recognition of Peronospora parasitica ) and ATR ( Arabidopsis thaliana recognized), respectively [2] . Six RPP loci have been cloned [3] . The corresponding recognized Hpa effectors have been identified for RPP1 , RPP5, RPP13 , and RPP39 , which recognize ATR1, ATR5, ATR13, and ATR39, respectively [4] , [5] , [6] , [7] . Many oomycetes including Hpa encode secreted proteins with an RxLR (or RxLR-EER) motif that is cleaved in the pathogen upon infection [8] . Previously, we defined a total of 475 Hpa gene models that encode effector candidates in the reference Hpa isolate Emoy2 [9] by applying the following criteria [10] : (1) proteins with a signal peptide and canonical RxLR motif, like ATR1, ATR13, and ATR39 (HaRxLs) [4] , [6] , [7] , reported by Baxter et al. [9] , (2) RxLR-like proteins with at least one non-canonical feature, like ATR5 (HaRxLLs) [5] , (3) putative Crinkler-like proteins with RxLR motif (HaRxLCRNs) [11] , (4) homologous proteins based on amino acid sequence similarity over the 5′ region including a signal peptide and RxLR motif (e.g., HaRxL1b, HaRxLL2b, and HaRxLCRN3b). In Arabidopsis Col-0, RPP4 confers resistance to Hpa isolates Emoy2 and Emwa1 [12] , but its cognate AVR effector gene(s) were not identified. We report here, using comparative genomics and transcriptomics among different isolates of Hpa , that the effector candidate HaRxL103 corresponds to the AVR gene. We also show that different Hpa resistance-breaking strains evade detection by RPP4 using two distinct mechanisms. Identification of RPP4 -recognized effectors Genome sequences and expression data during infection for Hpa Emoy2 and Waco9 were previously reported [9] , [10] . Here, we sequenced genomes of five other Hpa isolates (Emwa1, Cala2, Emco5, Maks9, and Hind2). 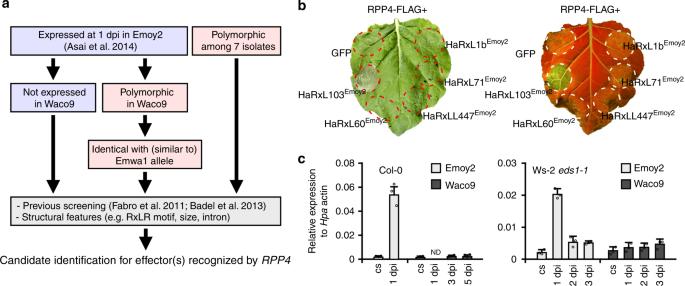Fig. 1 Identification of candidate effector(s) recognized byRPP4.aFlowchart to identify candidate effector(s) recognized byRPP4. InHpaeffectors expressed at 1 dpi inHpaEmoy2, not-expressed effectors inHpaWaco9 during infection and effectors that are polymorphic inHpaWaco9 and identical with or similar toHpaEmwa1 alleles were selected. Also,Hpaeffectors in which polymorphism among 7 differentHpaisolates are consistent with recognition phenotypes byRPP4were selected. After checking results in previous screening reported by Fabro et al.15and Badel et al.16and structural features, the candidates tested were identified.bHR cell death phenotypes when the candidates were co-expressed with RPP4 inN. benthamiana. The leaves inoculated withAgrobacteriumcontaining the indicated gene constructs were photographed at 3 dpi. The right one was photographed under UV to facilitate visualization of cell death.cExpression ofHaRxL103in conidiospores (cs) ofHpaEmoy2 and Waco9 and the infections in Arabidopsis Col-0 or Ws-2eds1-1mutant. The expression level was determined by qRT-PCR using specific primers forHaRxL103. Expression ofHpaactin was used to normalize the expression value in each sample. Data are means ± SDs from three biological replicates. ND not detectable As reported for other filamentous plant pathogens [13] , local biases were observed in the ratio of non-synonymous and synonymous nucleotide substitutions in predicted effector-encoding genes (Table 1 and Supplementary Data 1 and 2 ), suggesting that these genes might be under diversifying selection to evade recognition by cognate RPP genes. Of these seven Hpa isolates, Emoy2 and Emwa1 are recognized by Col-0 RPP4 [12] , [14] . In Hpa isolates, such as Waco9, that evade RPP4 detection, Hpa effector(s) recognized by RPP4 could be deleted, polymorphic, or not expressed. We investigated such possible variation with comparative genomics and transcriptomics, using transcriptome datasets of Hpa Emoy2 and Waco9 during infection [10] . In Hpa Emoy2-infected Arabidopsis Col-0 (an incompatible interaction), transcripts from Hpa clearly decreased from 1 day post-inoculation (dpi), consistent with Hpa Emoy2 growth being arrested upon recognition by RPP4 . The 65 predicted Hpa effectors expressed at 1 dpi in Hpa Emoy2 are thus strong candidates for an effector recognized by RPP4 . We also examined the genomes of seven sequenced Hpa isolates and analyzed transcriptome data of Hpa Waco9. These analyses revealed five candidate Hpa effectors [15] , [16] (Fig. 1a and Supplementary Data 3 ). HaRxL103 and HaRxL71 were prioritized because they were expressed at 1 dpi in Hpa Emoy2, but not expressed in Hpa Waco9, during infection. HaRxL60 and HaRxL1b were identical to alleles present in Hpa Emwa1, yet were found to be polymorphic in Hpa Waco9. HaRxLL447 was selected by identifying secreted proteins whose polymorphisms associated with recognition phenotypes among the seven sequenced Hpa isolates (Supplementary Fig. 1 ). Table 1 Number of synonymous and non-synonymous polymorphisms in Hpa isolates Full size table Fig. 1 Identification of candidate effector(s) recognized by RPP4 . a Flowchart to identify candidate effector(s) recognized by RPP4 . In Hpa effectors expressed at 1 dpi in Hpa Emoy2, not-expressed effectors in Hpa Waco9 during infection and effectors that are polymorphic in Hpa Waco9 and identical with or similar to Hpa Emwa1 alleles were selected. Also, Hpa effectors in which polymorphism among 7 different Hpa isolates are consistent with recognition phenotypes by RPP4 were selected. After checking results in previous screening reported by Fabro et al. [15] and Badel et al. [16] and structural features, the candidates tested were identified. b HR cell death phenotypes when the candidates were co-expressed with RPP4 in N. benthamiana . The leaves inoculated with Agrobacterium containing the indicated gene constructs were photographed at 3 dpi. The right one was photographed under UV to facilitate visualization of cell death. c Expression of HaRxL103 in conidiospores (cs) of Hpa Emoy2 and Waco9 and the infections in Arabidopsis Col-0 or Ws-2 eds1-1 mutant. The expression level was determined by qRT-PCR using specific primers for HaRxL103 . Expression of Hpa actin was used to normalize the expression value in each sample. Data are means ± SDs from three biological replicates. ND not detectable Full size image HaRxL103 Emoy2 is an Hpa effector recognized by RPP4 To identify effector(s) recognized by RPP4 , the five selected GFP-fused candidates were transiently co-expressed with FLAG-tagged RPP4 via Agrobacterium in leaves of Nicotiana benthamiana (Supplementary Fig. 2a ). GFP-HaRxL103 Emoy2 , but not GFP and the other GFP-fused candidates, induced RPP4 -dependent HR within 3 days (Fig. 1b ). We confirmed that HaRxL103 is expressed at 1 dpi in Hpa Emoy2, but not in Hpa Waco9, during infection on Arabidopsis Col-0 (Fig. 1c ). To evaluate the expression patterns of HaRxL103 in a compatible interaction, we inoculated Arabidopsis enhanced disease susceptibility 1 mutant Ws-2 eds1-1 with Hpa Emoy2 and Waco9. Ws-2 eds1-1 is susceptible to both Hpa Emoy2 and Waco9 [17] . HaRxL103 was induced at 1 dpi in Hpa Emoy2, but not in Hpa Waco9, during infection on Ws-2 eds1-1 (Fig. 1c ). RPP4 encodes an N-terminal TIR domain-containing NLR (TIR-NLR). As EDS1 is required for the function of TIR-NLR proteins [18] , we tested if EDS1 is required for RPP4 function. In N. benthamiana leaves in which the homolog of EDS1 , NbEDS1 , was transiently silenced by overexpressing hairpin RNA of NbEDS1 (NbEDS1-RNAi), estradiol-inducible GFP-HaRxL103 Emoy2 (Est-103 Emoy2 ) was co-expressed with RPP4-FLAG, and then GFP-HaRxL103 Emoy2 was induced by infiltration with estradiol. HR cell death induced by GFP-HaRxL103 Emoy2 and RPP4-FLAG co-expression was observed in a leaf area overexpressing hairpin RNA targeted against GUS (GUS-RNAi) as a control, whereas the HR cell death was compromised in NbEDS1 -silenced leaf area (Fig. 2a, b ). Fig. 2 HaRxL103 Emoy2 is recognized by RPP4 in an EDS1 -dependent manner. a N. benthamiana leaves were inoculated with Agrobacterium containing estradiol-inducible GFP-HaRxL103 Emoy2 (Est-103 Emoy2 ), RPP4-FLAG and GUS-RNAi or NbEDS1-RNAi constructs. The different inoculation sites were infiltrated with 20 μM estradiol (Est) or water (Mock) 24 h after the inoculation. The leaves were photographed under UV at 2 days after the infiltration. b Confirmation of proteins accumulation and NbEDS1 silencing. Total proteins and RNAs were prepared from N. benthamiana leaves described above 8 h after infiltration with estradiol or water. Immunoblot analyses were done using anti-GFP (top panel) and anti-FLAG (middle panel) antibodies. Protein loads were monitored by Coomassie Brilliant Blue (CBB) staining of the bands corresponding to ribulose-1,5-bisphosphate carboxylase (Rubisco) large subunit (bottom panel). The bar chart indicates expression levels of NbEDS1 determined by qRT-PCR. Data are means ± SDs from three technical replicates. The experiments were repeated two times with similar results. c In planta interaction between HaRxL103 Emoy2 and RPP4. Co-immunoprecipitation was performed with extracts from N. benthamiana leaves co-expressing GFP or GFP-HaRxL103 Emoy2 with RPP4-FLAG. MACS MicroBeads with GFP antibody were used for immunoprecipitation, and anti-GFP (upper panel) and anti-FLAG (lower panel) antibodies were used to detect the related proteins in the immunoprecipitates. Protein accumulation ( d ), AtPR1 expression ( e ), and Hpa growth ( f ) in Arabidopsis Col-0 and Col-0 rpp4 transgenic lines containing estradiol-inducible GFP (Est-GFP) and Est-103 Emoy2 constructs. d Total proteins and RNAs were prepared from 2-week old plants 24 h after spray treatment with 40 μM estradiol or water. Immunoblot analyses were done using anti-GFP as described in ( b ). Asterisks indicate the detected GFP or GFP-HaRxL103 Emoy2 constructs. e The expression level of AtPR1 was determined by qRT-PCR. Data are means ± SDs from three biological replicates. Different letters indicate significantly different values at p < 0.05 (one-way ANOVA, Tukey’s HSD). f Three-week-old transgenic lines 24 h after spray treatment with estradiol or water were inoculated with Hpa Waco9. Conidiospores were harvested and counted at 5 dpi. Data are means ± SEs from five biological replicates. Different letters indicate significantly different values at p < 0.01 (one-way ANOVA, Tukey’s HSD) Full size image We tested in planta interaction between GFP-HaRxL103 Emoy2 and RPP4-FLAG by co-immunoprecipitation (Fig. 2c and Supplementary Fig. 3 ). To test if HaRxL103 Emoy2 is recognized by RPP4 in Arabidopsis, we created transformants containing Est-103 Emoy2 and estradiol-inducible GFP (Est-GFP) as a control in Arabidopsis Col-0 or Col-0 rpp4 mutant (Fig. 2d ). As no visible HR cell death was observed after treatment with estradiol in the transformants, expression of PR1 , a defense marker gene, was investigated. Strong induction of PR1 was observed in Col-0 Est-103 Emoy2 , but not Col-0 Est-GFP, after treatment with estradiol, whereas Col-0 rpp4 Est-103 Emoy2 showed lower PR1 expression after the treatment compared to Col-0 Est-103 Emoy2 (Fig. 2e ). We tested if HaRxL103 Emoy2 induction in Col-0 could activate disease resistance against virulent Hpa Waco9. No Hpa Waco9 sporulation was observed on Col-0 Est-103 Emoy2 pretreated with estradiol (Fig. 2f ). These results indicate that HaRxL103 Emoy2 is recognized by RPP4 in an EDS1 -dependent manner. HaRxL103 Emoy2 recognition requires RPP4 nuclear localization To check in planta subcellular localization of HaRxL103 Emoy2 , GFP-HaRxL103 Emoy2 was transiently expressed in N. benthamiana leaves, and fluorescence was observed. Fluorescence signals were seen in cytoplasm and nucleus, and especially in the nucleolus (Supplementary Fig. 4a ). We evaluated which subcellular compartment HaRxL103 Emoy2 is essential for RPP4 -mediated recognition by expressing GFP-HaRxL103 Emoy2 attached to a nuclear export signal (NES), a nuclear localization signal (NLS), or mutated nes and nls sequences. The fluorescence signals from NES-fused and NLS-fused GFP-HaRxL103 Emoy2 were detected only in cytoplasm and nucleus, respectively, whereas mutated nes and nls ones showed similar fluorescence patterns to GFP-HaRxL103 Emoy2 (Supplementary Fig. 4a ). HR cell death by overexpression of GFP-NES-HaRxL103 Emoy2 , but not the other constructs, was compromised compared to that induced by GFP-HaRxL103 Emoy2 when co-expressed with RPP4-FLAG in N. benthamiana leaves (Supplementary Fig. 4b and c ). These results suggest that in planta nuclear localization of HaRxL103 Emoy2 is essential for recognition by RPP4 . Like HaRxL103 Emoy2 , RPP4 is localized to cytoplasm and nucleus [19] . To evaluate whether nuclear localization of RPP4 is essential for recognition of HaRxL103 Emoy2 , RPP4 fused to NES or nes (RPP4-NES and RPP4-nes, respectively) were constructed. As we could observe no fluorescent signals in plant cells expressing RPP4-GFP, fractionation of cytoplasmic and nuclear proteins was done to check in planta subcellular localization of RPP4-NES/nes. RPP4-FLAG and RPP4-nes-FLAG were detected in both cytoplasmic and nuclear fractions, whereas RPP4-NES-FLAG was detected only in a cytoplasmic fraction (Supplementary Fig. 5a ). RPP4-nes-FLAG induced HR cell death at the same levels as RPP4-FLAG, but HR cell death mediated by RPP4-NES-FLAG was compromised when co-expressed with GFP-HaRxL103 Emoy2 in N. benthamiana leaves (Supplementary Fig. 5b and c ). These results suggest that nuclear localization of RPP4 is important for recognition of HaRxL103 Emoy2 . HaRxL103 Hind2 evades recognition by changing localization In the seven genome-sequenced Hpa isolates, previous genetic studies revealed that Emoy2 and Emwa1, but not five other isolates, are recognized by RPP4 [12] , [14] . We investigated genetic diversity of HaRxL103 alleles among the seven Hpa isolates. The genomic sequence data showed that there are two non-synonymous nucleotide differences in the Waco9 and Cala2 alleles ( HaRxL103 Waco9/Cala2 ), one in the Emco5 and Maks9 alleles ( HaRxL103 Emco5/Maks9 ), and one in the Hind2 allele ( HaRxL103 Hind2 ) compared to the Emoy2 allele ( HaRxL103 Emoy2 ). Emwa1 ( HaRxL103 Emwa1 ) is heterozygous and carries both Emoy2 and Waco9/Cala2 alleles (Fig. 3a and Supplementary Fig. 6 ). We tested in planta subcellular localization and RPP4 -mediated HR cell death inducibility of HaRxL103 alleles. GFP-fused HaRxL103 alleles were transiently expressed with or without RPP4-FLAG in N. benthamiana . GFP-HaRxL103 Waco9/Cala2 and GFP-HaRxL103 Emco5/Maks9 were localized to cytoplasm and nucleus, especially nucleolus, as observed for GFP-HaRxL103 Emoy2 , whereas we observed only a weak fluorescent signal of GFP-HaRxL103 Hind2 in the nucleolus (Fig. 3b ; top). Their subcellular localization was unaltered by co-expression with RPP4-FLAG (Fig. 3b ; bottom). GFP-HaRxL103 Waco9/Cala2 and GFP-HaRxL103 Emco5/Maks9 induced HR cell death indistinguishable from GFP-HaRxL103 Emoy2 when transiently co-expressed with RPP4-FLAG in N. benthamiana , but HR cell death induced by GFP-HaRxL103 Hind2 was dramatically reduced (Fig. 3c ). In Col-0 transformants containing estradiol-inducible GFP-HaRxL103 Emoy2 (Est-103 Emoy2 ) and GFP-HaRxL103 Hind2 (Est-103 Hind2 ), similar fluorescent signal patterns to ones in N. benthamiana transiently expressed were observed (Fig. 3b, d, and e ). Consistent with HR phenotypes in N. benthamiana , Col-0 Est-103 Hind2 showed less induction of PR1 than Col-0 Est-103 Emoy2 after treatment with estradiol (Fig. 3f ). Hpa sporulated on Col-0 Est-103 Hind2 , but not on Col-0 Est-103 Emoy2 , pretreated with estradiol (Fig. 3g ). Fig. 3 Effect of mutations in HaRxL103 alleles on in planta subcellular localization and recognition by RPP4 . a Schematic structures of HaRxL103 alleles. Filled and diagonal boxes indicate an N-terminal signal peptide and an RxLR motif, respectively. Red-letter residues indicate polymorphic sites. E, Glu; H, His; R, Arg; D, Asp; K, Lys; Q, Gln. b Subcellular localization of HaRxL103 alleles. GFP-tagged HaRxL103 alleles were transiently (co)expressed with/without RPP4-FLAG via agroinfiltration in N. benthamiana . Images are from GFP channel and single-plane confocal images. Scale bars, 10 μm. c HR cell death phenotypes when co-expressed of HaRxL103 alleles with RPP4 in N. benthamiana . The leaves inoculated with Agrobacterium containing the indicated gene constructs were photographed under UV at 3 dpi. Protein accumulation ( d ), subcellular localization ( e ), AtPR1 expression ( f ), and Hpa growth ( g ) in Arabidopsis Col-0 transgenic lines containing Est-GFP, Est-103 Emoy2 and estradiol-inducible GFP-HaRxL103 Hind2 (Est-103 Hind2 ) constructs. Immunoblot, qRT-PCR and Hpa growth analyses were done as described in Fig. 2d–f . d Asterisks indicate the detected GFP, GFP-HaRxL103 Emoy2 or GFP-HaRxL103 Hind2 constructs. e Col-0 transgenic lines pretreated with estradiol were DAPI-stained. The upper image is from the GFP channel, the middle image is from the DAPI channel, and the lower image is the overlay of the GFP and DAPI channels. Scale bars, 10 μm. f Data are means ± SDs from three biological replicates. Different letters indicate significantly different values at p < 0.01 (one-way ANOVA, Tukey’s HSD). g Data are means ± SEs from five biological replicates. Different letters indicate significantly different values at p < 0.01 (one-way ANOVA, Tukey’s HSD) Full size image The finding that GFP-HaRxL103 Hind2 shows little accumulation in nucleolus and less inducibility in RPP4 -mediated HR cell death than GFP-HaRxL103 Emoy2 prompted us to examine the possibility that reduced recognition of HaRxL103 Hind2 by RPP4 is due to the difference in subcellular localization. To test this hypothesis, NLS- and the mutated nls-fused GFP-HaRxL103 Hind2 derivatives (GFP-NLS-HaRxL103 Hind2 and GFP-nls-HaRxL103 Hind2 , respectively) were constructed. For the subcellular localization assay, RFP-fused HaRxL44 Emoy2 , an Hpa effector that localizes to the plant cell nucleolus [20] , was co-expressed as a nucleolus marker. We observed nucleolar localization of GFP-NLS-HaRxL103 Hind2 similar to GFP-HaRxL103 Emoy2 , whereas little accumulation of GFP-nls-HaRxL103 Hind2 was observed in nucleolus as for GFP-HaRxL103 Hind2 (Fig. 4a ). Importantly, GFP-NLS-HaRxL103 Hind2 , but not GFP-nls-HaRxL103 Hind2 , induced HR cell death at the same level as GFP-HaRxL103 Emoy2 when co-expressed with RPP4-FLAG in N. benthamiana (Fig. 4b ). Fig. 4 The mutation in HaRxL103 Hind2 affects in planta subcellular localization. a Subcellular localization of GFP-HaRxL103 Emoy2 (GFP-103 Emoy2 ), GFP-HaRxL103 Hind2 , and NLS- or nls-fused GFP-HaRxL103 Hind2 . GFP-tagged HaRxL103 Emoy2 and HaRxL103 Hind2 variants were transiently co-expressed with RFP-HaRxL44 Emoy2 via agroinfiltration in N. benthamiana . The upper image is from the GFP channel, the middle image is from the RFP channel, and the lower image is the overlay of the GFP and RFP channels. Fluorescence intensity profile (GFP, green; RFP, red) across the white arrow was performed using the analyzing software (Leica, bottom). Scale bars, 10 μm. b HR cell death phenotypes when co-expressed of HaRxL103 Emoy2 and HaRxL103 Hind2 variants with RPP4 in N. benthamiana . The leaves inoculated with Agrobacterium containing the indicated gene constructs were photographed under UV at 3 dpi. c A predicted NLS sequence from HaRxL103 Emoy2 and HaRxL103 Hind2 . Prediction of NLS in HaRxL103 Emoy2 or HaRxL103 Hind2 was done in cNLS Mapper. Position of predicted NLS and score for the prediction are indicated. Identical sequences are indicated in white on black. d Subcellular localization of GFP-fused predicted NLS from HaRxL103 Emoy2 (NLS Emoy2 ) and HaRxL103 Hind2 (NLS Hind2 ). GFP, GFP-NLS Emoy2 , and GFP-NLS Hind2 were transiently co-expressed with RFP-HaRxL44 Emoy2 via agroinfiltration in N. benthamiana . Imaging was performed as described in ( a ). Scale bars, 10 μm Full size image The prediction of NLS revealed that the non-synonymous single nucleotide variant (SNV) in HaRxL103 Hind2 is in a predicted mono-partite NLS, and the amino acid sequence in HaRxL103 Hind2 no longer corresponds to a predicted NLS (Fig. 4c and Supplementary Fig. 6 ). To evaluate if the predicted NLS is functional and if the mutation in HaRxL103 Hind2 affects the function, GFP fusions to the predicted NLS sequences from HaRxL103 Emoy2 and HaRxL103 Hind2 (GFP-NLS Emoy2 and GFP-NLS Hind2 , respectively) were constructed. GFP-NLS Emoy2 was visible in nucleoplasm and the nucleolus as observed for RFP-HaRxL44 Emoy2 , a nucleolus-localizing Hpa effector [20] , whereas GFP-NLS Hind2 showed nuclear-cytoplasmic localization and little nucleolar localization compared to GFP-NLS Emoy2 (Fig. 4d ), suggesting that the predicted NLS from HaRxL103 Emoy2 , but not HaRxL103 Hind2 , functions as an NLS. These results indicate that the mutation in HaRxL103 Hind2 alters in planta subcellular localization, resulting in evasion of recognition by RPP4 . Localization of HaRxL103-RPP4 interaction The requirement of HaRxL103 Emoy2 for nuclear localization to be recognized by RPP4 (Fig. 4 and Supplementary Fig. 4 ) indicates the possibility that HaRxL103 Emoy2 interacts with RPP4 in nucleus. To test this hypothesis, we performed bimolecular fluorescence complementation analysis by co-expressing nVenus/cCFP-HaRxL103 Emoy2 with RPP4-nVenus/cCFP in all combinations, but we failed to observe fluorescent signals. Therefore, co-immunoprecipitation in a nuclear fraction was performed. Cytoplasmic and nuclear protein extracts were separately isolated from N. benthamiana leaves transiently expressing GFP-HaRxL103 Emoy2 and RPP4-FLAG. Co-immunoprecipitation assays in cytoplasmic and nuclear fractions revealed HaRxL103 Emoy2 -RPP4 interaction in both cytoplasm and nucleus (Fig. 5a ). We also checked whether GFP-HaRxL103 Hind2 and NLS/nls-fused GFP-HaRxL103 Hind2 interact with RPP4-FLAG in cytoplasm and/or nucleus (Fig. 5b–d ). GFP-HaRxL103 Hind2 and GFP-nls-HaRxL103 Hind2 were detected only in cytoplasmic fractions, whereas GFP-NLS-HaRxL103 Hind2 was detected only in nuclear fractions. We confirmed in planta interaction of GFP-HaRxL103 Hind2 and GFP-NLS/nls-HaRxL103 Hind2 with RPP4-FLAG in each fraction, suggesting that the mutation in HaRxL103 Hind2 does not affect the interaction with RPP4. Fig. 5 Interactions between HaRxL103 Emoy2 /HaRxL103 Hind2 and RPP4 in cytoplasm and/or nucleus. In planta interaction of GFP-HaRxL103 Emoy2 ( a ), GFP-HaRxL103 Hind2 ( b ), and GFP-NLS/nls-HaRxL103 Hind2 ( c , d ) with RPP4-FLAG in cytoplasm and nucleus. Cytoplasmic (C) and nuclear (N) protein extracts were separately isolated from N. benthamiana leaves inoculated with Agrobacterium containing the indicated gene constructs at 2 dpi. Co-immunoprecipitation was performed with each extract using MACS MicroBeads with GFP antibody. Anti-GFP (upper panel), anti-FLAG (the 2nd panel), anti-UGPase (the 3rd panel), and anti-Histone H3 antibodies (bottom panel) were used to detect the related proteins in the immunoprecipitates. UGPase and Histone H3 were checked as markers for cytoplasmic and nuclear proteins, respectively Full size image Virulence co-segregates with lack of HaRxL103 expression Hpa isolates Waco9, Cala2, Emco5, and Maks9 also avoid recognition by RPP4 , but HaRxL103 Waco9/Cala2 and HaRxL103 Emco5/Maks9 activate RPP4 -dependent HR cell death in N. benthamiana (Fig. 3c ). We tested if these Hpa isolates evade RPP4 -mediated immunity through lack of HaRxL103 expression, and found HaRxL103 is not expressed in Hpa Waco9, but is in Emoy2, during infection (Fig. 1c ). Previously, an outcrossed F2 population of Hpa isolates Emoy2 and Maks9 was used to identify Hpa recognized effector genes for six known R genes including RPP4 [21] . Positional cloning using the Emoy2/Maks9 F2 progeny identified ATR1 , ATR5 , and ATR13 as Hpa AVR genes recognized by RPP1 , RPP5 , and RPP13 , respectively [4] , [5] , [6] . In the Emoy2/Maks9 F2 progeny, segregation data for the Hpa gene locus corresponding with recognition by RPP4 ( ATR4 ) revealed that RPP4 -mediated immunity is controlled by a semi-dominant allele at a single locus [21] . To evaluate whether the HaRxL103 locus is linked to RPP4 -mediated immunity in the Emoy2/Maks9 F2 progeny, we designed a CAPS (cleaved amplified polymorphic sequence) marker based on polymorphism between Emoy2 and Maks9 HaRxL103 alleles. The HaRxL103 locus was unlinked to RPP4 -dependent recognition in the Emoy2/Maks9 F2 progeny (Supplementary Table 1 ). Conceivably, the genetically defined ATR4 gene regulates expression of HaRxL103 . We created an outcrossed progeny of Hpa isolates Emoy2 and Cala2, and checked phenotypes on Arabidopsis CW84, an Hpa susceptible recombinant inbred line generated from a cross between Col-0 and Ws-2 [22] , and on CW84 lines carrying transgenic RPP4 (CW84:RPP4 Col ) [12] . The Emoy2/Cala2 F1 Hpa showed avirulence on CW84:RPP4 Col as observed for Emoy2 (Supplementary Fig. 7 ), whereas the F2 progeny segregated with virulent or avirulent phenotypes on CW84:RPP4 Col . Arabidopsis Ws-2 eds1-1 mutant [17] was susceptible to all the Emoy2/Cala2 F2 progeny. We checked the expression levels of HaRxL103 in the individual F2 progeny by qRT-PCR at 2 and 4 dpi on Ws-2 eds1-1 . In all F2 progeny which showed avirulence on CW84:RPP4 Col , HaRxL103 expression was observed during at least one time point, whereas no expression was observed in virulent isolates (Fig. 6a ). Genotyping using a CAPS marker designed to detect polymorphism between Emoy2 and Cala2 HaRxL103 alleles revealed segregation of the HaRxL103 locus in virulent isolates (Fig. 6b ). These results suggest that virulence correlates with lack of HaRxL103 expression, but does not map to the HaRxL103 locus in an Emoy2/Cala2 F2. Fig. 6 In an Emoy2/Cala2 F2, virulence consists with lack of HaRxL103 expression. a Expression of HaRxL103 during infection in Emoy2/Cala2 F2 individual progeny which showed virulence or avirulence on CW84:RPP4 Col plants. Total RNA was prepared from the infections in Arabidopsis Ws-2 eds1-1 mutant at 2 or 4 dpi. qRT-PCR analysis was done as described in Fig. 1c . b Genotyping of the HaRxL103 locus in Emoy2/Cala2 F2 individual progeny which showed virulence on CW84:RPP4 Col plants. Genotyping of the HaRxL103 locus was performed by a CAPS (cleaved amplified polymorphic sequence) method. Upper and bottom panels indicate PCR products and those after restriction enzyme (RE) treatment, respectively. M marker, ND not detectable Full size image We report here the identification of HaRxL103, an Hpa effector recognized by Arabidopsis RPP4 , and two modes of evasion of recognition in different resistance-breaking strains of Hpa . Of seven sequenced Hpa isolates, Emoy2 and Emwa1 are avirulent on Arabidopsis genotypes containing functional RPP4 , whereas Waco9, Cala2, Emco5, Maks9, and Hind2 evade recognition by RPP4 [12] , [14] . Co-expression of HaRxL103 Emoy2 with RPP4 resulted in HR cell death in N. benthamiana in an NbEDS1 -dependent manner, and ectopic expression of HaRxL103 Emoy2 induced immune responses in Col-0 plants containing RPP4 . Co-immunoprecipitation analysis revealed that HaRxL103 Emoy2 interacts with RPP4 in both cytoplasm and nucleus. We found that nuclear, and perhaps nucleolar, localization of HaRxL103 Emoy2 is required to trigger RPP4 -mediated immune responses and that the Hpa isolate Hind2 evades RPP4 recognition by a mutation in a functional NLS in HaRxL103. In contrast, Hpa isolates Waco9 and Cala2 evade recognition by RPP4 through lack of HaRxL103 expression. Finally, analyses in Emoy2/Cala2 F2 individual progeny showing virulence or avirulence on CW84:RPP4 Col revealed that virulence is associated with lack of HaRxL103 expression, but that this lack of expression is conferred by a gene that is not linked to the HaRxL103 locus. During co-evolution with plants, pathogens have inactivated deleterious genes, including recognized effector genes, by diverse mechanisms such as gene loss, mutation, and gene silencing. In filamentous plant pathogens, such as Hpa and Phytophthora species, genes encoding putative effector proteins (e.g., RxLR effectors) show signatures of diversifying selection [9] , [13] , [23] . In this study, we confirmed this correlation in Hpa isolates (Table 1 and Supplementary Data 1 and 2 ). Hpa Waco9 evades recognition by Arabidopsis R gene RPP1 through loss of its cognate recognized effector ATR1 from its genome [10] . Virulent isolates of wheat stem rust break resistance conferred by the wheat Sr35 resistance gene through loss of AvrSr35 by the insertion of a mobile element [24] . ATR1 and ATR13 are extremely polymorphic and this allelic diversity enables evasion of recognition by specific alleles of their corresponding R genes, RPP1 and RPP13 [4] , [6] , [25] , [26] . In Phytophthora sojae , a key amino acid mutation in PsAvr3c impairs a physical association with the host protein GmSKRPs involved in Rps3c -mediated soybean immunity, resulting in evasion of recognition by Rps3c [27] , [28] . There are some non-synonymous SNVs among HaRxL103 alleles (Fig. 3a and Supplementary Fig. 6 ). We identified a single point mutation in the Hind2 allele ( HaRxL103 Hind2 ) that is located in a functional NLS within HaRxL103, resulting in exclusion of the protein from the nucleus (at least nucleolus), that correlates with evasion of RPP4 -mediated immune responses (Figs. 3 and 4 ). This conclusion is supported by the finding that the fusion of NLS to HaRxL103 Hind2 could restore HR cell death triggered by co-expression with RPP4 (Fig. 4b ). In this study, GFP-tagged proteins were ectopically overexpressed to check those subcellular localizations. Although we cannot rule out the possibility that the localization of GFP-tagged HaRxL103 does not reflect the real localization of native HaRxL103 proteins during Hpa infection, in planta subcellular localization of HaRxL103 correlated with RPP4 -mediated immunity in the conditions tested. This is, to our knowledge, the first report that a pathogen effector can avoid recognition by its cognate R gene through changing subcellular localization in host cells. Transcriptional silencing of AVR effector genes to evade resistance in host plants containing their cognate R genes has also been reported in Phytophthora species [29] . Qutob et al. [30] demonstrated transgenerational gene silencing of P. sojae Avr3a . Although the mechanisms responsible for its establishment remain to be determined, they found an association between small RNA accumulation and gene silencing at the Avr3a locus. Interestingly, comparative genomics among Phytophthora species revealed that RxLR effector-rich regions are enriched for genes related to epigenetic processes, suggesting a potential role for epigenetic mechanisms in oomycete pathogen evolution [23] . Despite carrying non-synonymous polymorphisms from HaRxL103 Emoy2 , the HaRxL103 Waco9/Cala2 and HaRxL103 Emco5/Maks9 alleles cause RPP4 -dependent HR cell death comparable to HaRxL103 Emoy2 in N. benthamiana (Fig. 3a, c ). We infer that Hpa isolates Waco9, Cala2, Emco5, and Maks9 evade RPP4 -mediated immunity through loss of HaRxL103 expression. Consistent with this model, HaRxL103 is induced during infection in Hpa Emoy2, but not in Waco9 (Fig. 1c ), and virulence co-segregates with lack of HaRxL103 expression in an Emoy2/Cala2 F2 (Fig. 6a ). Interestingly, 2 kb upstream and 0.5 kb downstream of the HaRxL103 -coding regions are identical between Emoy2 and Waco9, suggesting that expression of HaRxL103 could be regulated by epigenetic mechanisms and/or specific transcriptional regulator(s) for Hpa isolates (discussed in the section below). The gene-for-gene model predicts the outcome of interactions between Arabidopsis accessions and Hpa isolates [2] . ATR4 was originally defined as an Hpa gene locus associated with the RPP4 -mediated immunity in an Emoy2-Maks9 F2 [21] . In this study, we revealed that HaRxL103 triggers RPP4 -mediated immunity, but there is no genetic linkage between the HaRxL103 locus and RPP4 -mediated immunity in the Emoy2/Maks9 F2 progeny or in the Emoy2/Cala2 F2 progeny. We propose referring to HaRxL103 Emoy2 as AvrRPP4, but not ATR4. We suggest ATR4 should be reserved for the locus at which genetic variation is found that regulates HaRxL103 expression. The flanking sequence of the HaRxL103 -coding region is identical in Hpa virulent isolate Waco9 and avirulent isolate Emoy2, so we propose that allelic variation between virulent and avirulent isolates is found in gene(s) involved in epigenetic and/or transcriptional regulation of HaRxL103 . In flax rust, “inhibitor genes” for avirulence have also been identified [31] ; this might also reflect allelic variation in a transcriptional regulator that controls expression of a recognized effector. Further analysis by positional cloning is required to uncover ATR4 . Effector genes that trigger ETI on their host plants are likely to be rapidly lost unless they contribute to virulence on susceptible host plants. Both ATR1 and ATR13 trigger ETI on plants that carry RPP1 and RPP13 , respectively, but promote virulence in a compatible interaction [32] . To evaluate whether HaRxL103 Emoy2 has a virulence function, we measured Hpa growth on Col-0 rpp4 Est-GFP and Col-0 rpp4 Est-103 Emoy2 . Although Hpa sporulates on Col-0 rpp4 Est-103 Emoy2 pretreated with estradiol, Hpa growth is reduced compared to non-estradiol-treated Col-0 rpp4 Est-103 Emoy2 (Supplementary Fig. 8a and b ), suggesting that HaRxL103 Emoy2 might still be weakly recognized in a Col-0 rpp4 mutant. Consistent with this, although PR1 expression is much more strongly induced in Col-0 Est-103 Emoy2 than in Col-0 rpp4 Est-103 Emoy2 , PR1 expression is still weakly induced in Col-0 rpp4 Est-103 Emoy2 after treatment with estradiol (Fig. 2e ). Hpa Emoy2 sporulates on Col-0 rpp4 , but grows better on Col-0 eds1-2 , whereas Hpa Waco9, in which HaRxL103 is not expressed, is equally virulent on Col-0, Col-0 rpp4 , and Col-0 eds1-2 (Fig. 1c and Supplementary Fig. 8c ). As HaRxL103 Emoy2 still induces some immune responses in Col-0 rpp4 , we could not assess the virulence function. Loss-of-function analysis of HaRxL103 in Hpa is not currently technically feasible. If HaRxL103 Emoy2 has a virulence function, it would be interesting to investigate whether HaRxL103 Hind2 still has that function. In planta subcellular localization analysis revealed reduced accumulation of HaRxL103 Hind2 in the nucleolus compared to HaRxL103 Emoy2 (Fig. 3b ). Fusion of NLS to HaRxL103 Hind2 restored accumulation in nucleolus and complemented the loss of induction of RPP4 -mediated immunity (Fig. 4a, b ). In addition, co-immunoprecipitation analysis revealed the interaction of HaRxL103 Emoy2 and HaRxL103 Hind2 with RPP4 in cytoplasm and/or nucleus (Fig. 5 ). Exclusion of HaRxL103 from the nucleus abolished RPP4 -mediated HR cell death (Supplementary Fig. 3 ). These results suggest that the HaRxL103-RPP4 interaction in the nucleus (perhaps nucleolus) is essential for induction of RPP4 -mediated immunity. Although the host target of HaRxL103 remains to be defined, we hypothesize that HaRxL103 exerts its virulence function in the host nucleus, and perhaps in the nucleolus. HaRxL103 Hind2 might therefore lose virulence function. The nucleolus is the site for ribosomal RNA synthesis and ribosome assembly. Recent studies revealed a role for the nucleolus in the control of various tumor suppressors and oncogenes [33] . Investigation of the HaRxL103 function might enable unknown functions of the nucleolus to be revealed. Plant material and growth Arabidopsis plants were grown at 22 °C under a 10-h photoperiod and a 14-h dark period in environmentally controlled growth cabinets. N. benthamiana plants were grown at 25 °C under a 16-h photoperiod and an 8-h dark period in environmentally controlled growth cabinets. For Col-0 rpp4 mutant, we used a homozygous line from the SALK named SALK017569 [34] . 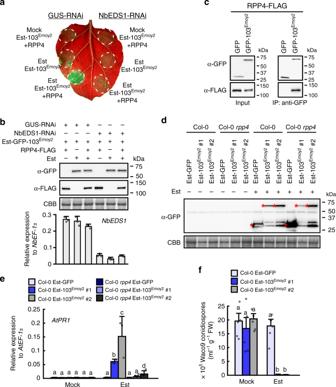Fig. 2 HaRxL103Emoy2is recognized byRPP4in anEDS1-dependent manner.aN. benthamianaleaves were inoculated withAgrobacteriumcontaining estradiol-inducible GFP-HaRxL103Emoy2(Est-103Emoy2), RPP4-FLAG and GUS-RNAi or NbEDS1-RNAi constructs. The different inoculation sites were infiltrated with 20 μM estradiol (Est) or water (Mock) 24 h after the inoculation. The leaves were photographed under UV at 2 days after the infiltration.bConfirmation of proteins accumulation andNbEDS1silencing. Total proteins and RNAs were prepared fromN. benthamianaleaves described above 8 h after infiltration with estradiol or water. Immunoblot analyses were done using anti-GFP (top panel) and anti-FLAG (middle panel) antibodies. Protein loads were monitored by Coomassie Brilliant Blue (CBB) staining of the bands corresponding to ribulose-1,5-bisphosphate carboxylase (Rubisco) large subunit (bottom panel). The bar chart indicates expression levels ofNbEDS1determined by qRT-PCR. Data are means ± SDs from three technical replicates. The experiments were repeated two times with similar results.cIn planta interaction between HaRxL103Emoy2and RPP4. Co-immunoprecipitation was performed with extracts fromN. benthamianaleaves co-expressing GFP or GFP-HaRxL103Emoy2with RPP4-FLAG. MACS MicroBeads with GFP antibody were used for immunoprecipitation, and anti-GFP (upper panel) and anti-FLAG (lower panel) antibodies were used to detect the related proteins in the immunoprecipitates. Protein accumulation (d),AtPR1expression (e), andHpagrowth (f) in Arabidopsis Col-0 and Col-0rpp4transgenic lines containing estradiol-inducible GFP (Est-GFP) and Est-103Emoy2constructs.dTotal proteins and RNAs were prepared from 2-week old plants 24 h after spray treatment with 40 μM estradiol or water. Immunoblot analyses were done using anti-GFP as described in (b). Asterisks indicate the detected GFP or GFP-HaRxL103Emoy2constructs.eThe expression level ofAtPR1was determined by qRT-PCR. Data are means ± SDs from three biological replicates. Different letters indicate significantly different values atp< 0.05 (one-way ANOVA, Tukey’s HSD).fThree-week-old transgenic lines 24 h after spray treatment with estradiol or water were inoculated withHpaWaco9. Conidiospores were harvested and counted at 5 dpi. Data are means ± SEs from five biological replicates. Different letters indicate significantly different values atp< 0.01 (one-way ANOVA, Tukey’s HSD) A T-DNA insertion was checked by PCR using T-DNA left border primer (LBb1.3) and gene-specific primers (LP and RP) listed in Supplementary Table 2 . Previously published Arabidopsis lines were: Ws-2 eds1-1 17 , CW84 [12] , CW84:RPP4 Col,12 , and Col-0 eds1-2 [35] . Pathogen assays Hpa inoculation was done as described in Asai et al. [36] . Briefly, Arabidopsis plants were spray-inoculated to saturation with a spore suspension of 1 × 10 5 conidiospores/ml. Plants were covered with a transparent lid to maintain high humidity (90–100%) conditions in a growth cabinet at 16 °C under a 10-h photoperiod until the day for sampling. To evaluate conidiospore production, 5 pools of 3 plants for each Arabidopsis line were harvested in 1 ml of water. After vortexing, the amount of conidiospores released was determined using a haemocytometer. Genome sequencing and comparative genomics of Hpa isolates Genomic DNA was extracted from Hpa conidiospores using a Nucleon PhytoPure DNA extraction kit (GE Healthcare) according to the procedure of the manufacturer. 36 and 76 bp paired-end libraries were prepared using the Illumina TruSeq protocol and sequenced on an Illumina Genome Analyzer II. The reads were aligned to the Hpa Emoy2 v8.3 [9] using BWA [37] version 0.5.8. Trailing nucleotides with a quality score of less than 10 were trimmed using the -q option. In order to maximize the number of aligned reads, unaligned reads were re-aligned using Stampy [38] . SAMtools [39] version 0.1.18 was used to generate BAM files. Genetic variations between Hpa Emoy2 and each of the genome-sequenced isolates were predicted using SAMtools [39] version 0.1.18. Polymorphisms detailed in Table 1 and Supplementary Data 1 and 2 were filtered to have a minimum quality score of 10, depth of 20 and maximum depth of 500. These variant calls, including indels, were fed into SnpEff [40] version 3.2 which predicted the effect of polymorphisms to each Hpa Emoy2 gene in each sequenced isolate, which could then be sorted into those encoding synonymous and non-synonymous changes. To predict recognized effector candidates by association, homozygous polymorphisms were first compared across isolates using PileLine [41] version 1.2, and then selected according to the known pattern of recognition. For example, to identify RPP4 -recognized effector candidates, genes encoding secreted proteins with polymorphisms encoding non-synonymous changes in all isolates except Emoy2 and Emwa1 were queried. Polymorphisms were visualized and confirmed in BAM files with the Integrative Genomics Viewer [42] . Finally, to generate predicted sequences from each isolate, the Hpa Emoy2 v8.3 genome sequence [9] was corrected by substituting SNVs using a custom Perl script. Plasmid construction For transient gene expression in N. benthamiana , HaRxL103 Emoy2 (21–401 aa), HaRxL60 Emoy2 (20–202 aa), HaRxL1b Emoy2 (27–239 aa), HaRxL71 Emoy2 (20–466 aa), HaRxLL447 Emoy2 (21–112 aa), and HaRxL103 alleles (21–401 aa) without signal peptide sequence were cloned and assembled (using pENTR and Gateway System) into binary vector pK7WGF2 (with 35S promoter and N-terminal GFP fusion tag) [43] . The SV40 large T-antigen NLS (PKKKRKVGG) [44] or nls (PKAAAKVGG) and NES (NELALKLAGLDINK) [45] or nes (NELALKAAGADANK) were introduced into 5′ of HaRxL103 Emoy2 (21–401 aa) and HaRxL103 Hind2 (21–401 aa) by PCR using specific oligonucleotides coding for NLS/nls and NES/nes and assembled similarly into pK7WGF2. To generate RPP4-FLAG, fragments of RPP4 were amplified from Col-0 gDNA for Golden Gate assembly [46] , [47] into binary vector pICH86988 (with 35S promoter and C-terminal FLAG fusion tag). To generate RPP4-NES/nes-FLAG, NES (NELALKLAGLDINK) [45] or nes (NELALKAAGADANK) were introduced into 3′ of RPP4 by PCR using specific oligonucleotides coding for NES/nes and assembled similarly into pICH86988. To generate GFP-NLS Emoy2 and GFP-NLS Hind2 , both forward and reverse specific oligonucleotides coding for NLS Emoy2 (NRRKRRMFRY) and NLS Hind2 (NRQKRRMFRY) were designed and annealed by a temperature gradient from 95 °C to 25 °C. The annealed dsDNA of NLS Emoy2 and NLS Hind2 were assembled similarly into binary vector pICSL86955 (with 35S promoter, N-terminal GFP fusion tag). Prediction of NLS was done by cNLS Mapper [ http://nls-mapper.iab.keio.ac.jp/cgi-bin/NLS_Mapper_form.cgi ]. RPS4-FLAG construct was previously reported [48] . For transient silencing in N. benthamiana , pHellsgate8-GUS [49] was used as a control. To generate EDS1-RNAi, sense and anti-sense sequences specific for NbEDS1 and PDK intron sequence were amplified from N. benthamiana gDNA and pHellsgate vector, respectively, for Golden Gate assembly [46] , [47] into binary vector pICSL86977 (with 35S promoter) in the order; sense NbEDS1 fragment, PDK intron sequence, and anti-sense NbEDS1 fragment. For estradiol-inducible constructs, GFP-HaRxL103 Emoy2 and GFP-HaRxL103 Hind2 were amplified from pK7WGF2-GFP-HaRxL103 Emoy2 and pK7WGF2-GFP-HaRxL103 Hind2 , respectively, for Golden Gate assembly [46] , [47] into binary vector pICSL86933 (with 35S promoter fused to the LexA operator) containing a chimeric transcription activator XVE [50] . Transient gene expression and plant transformation For transient gene expression analysis, Agrobacterium tumefaciens strain AGL1 was used to deliver respective transgenes in N. benthamiana leaves, using methods previously described [51] . For co-expression, all bacterial suspensions carrying individual constructs were adjusted to OD 600 = 0.5 in the final mix for infiltration. Background of leaf images in Figs. 1b , 2a , 3c , and 4b and Supplementary Figs. 4b and 5c were removed by using Adobe Photoshop Elements 15. Unprocessed leaf images are provided as a Source Data file. For plant transformation, Arabidopsis Col-0 plant and Col-0 rpp4 mutant were transformed using the dipping method [52] . Briefly, flowering Arabidopsis plants were dipped with A. tumefaciens carrying a plasmid of interest, and the seeds were harvested to select the T1 transformants on selective MS media. T1 plants were checked for expression of the construct of interest by western blotting analysis. T2 seeds were sown on selective MS media, and the proportion of resistant versus susceptible plants was counted in order to identify lines with single T-DNA insertion. Transformed plants were transferred to soil and seeds collected. Two independent T3 homozygous lines were analyzed. RNA extraction, cDNA synthesis, and qRT-PCR Total RNAs were extracted using RNeasy Plant Mini Kit (Qiagen) according to the procedure of the manufacturer. Total RNAs (1 μg) were used for generating cDNAs in a 20 μl volume reaction according to Invitrogen Superscript III Reverse Transcriptase protocol. The obtained cDNAs were diluted five times, and 1 μl was used for 10 μl qPCR reaction. qPCR was performed in 10 μl final volume using 5 μl SYBR Green mix (Toyobo), 1 μl diluted cDNAs, and primers. qPCR was run on Mx3000P qPCR System (Agilent) using the following program: (1) 95 °C, 3 min; (2) [95 °C, 30 s, then 60 °C, 30 s, then 72 °C, 30 s] × 45, (3) 95 °C, 1 min followed by a temperature gradient from 55 to 95 °C. The relative expression values were determined using the comparative cycle threshold method (2 −ΔΔCt ). Hpa Actin , AtEF-1α , and NbEF1α were used as reference genes for Hpa infections, Arabidopsis and N. benthamiana , respectively. Primers used for qPCR are listed in Supplementary Table 2 . Protein extraction, immunoprecipitation, and nuclear extraction Leaves were ground to fine powder in liquid nitrogen and thawed in extraction buffer (50 mM Tris–HCl, pH 7.5, 150 mM NaCl, 10% glycerol, 10 mM DTT, 10 mM EDTA, 1 mM NaF, 1 mM Na 2 MoO 4 ·2H 2 O, 1% IGEPAL CA-630 from Sigma-Aldrich and 1% protease inhibitor cocktail from Sigma-Aldrich). Samples were cleared by centrifugation at 16,000 g for 15 min at 4 °C, and the supernatant was used for total protein extracts. GFP-fused and FLAG-fused proteins were detected by anti-GFP antibody (ab290; Abcam plc) in 1:8000 dilution and anti-FLAG antibody (A8592; Sigma-Aldrich) in 1:20,000 dilution, respectively. Immunoprecipitation was performed using μMACS GFP isolation kit and μMACS DYKDDDDK isolation kit according to the manufacturer’s instructions (Miltenyi Biotec). Nuclear extraction was done by a modified method based on that described by Xu et al. [53] . Approximately 30 g of N. benthamiana leaves was frozen in liquid nitrogen, ground to a fine powder and homogenized in 30 ml lysis buffer (20 mM Tris–HCl, pH 7.4, 25% glycerol, 20 mM KCl, 2 mM EDTA, 2.5 mM MgCl 2 , 250 mM sucrose, 10 mM DTT, 1 mM PMSF and protease inhibitor cocktail from Sigma-Aldrich). The homogenate was sequentially filtered through a nylon mesh. 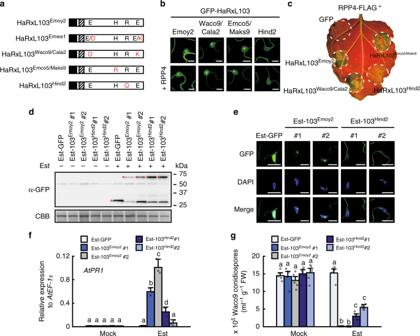Fig. 3 Effect of mutations in HaRxL103 alleles on in planta subcellular localization and recognition byRPP4.aSchematic structures of HaRxL103 alleles. Filled and diagonal boxes indicate an N-terminal signal peptide and an RxLR motif, respectively. Red-letter residues indicate polymorphic sites. E, Glu; H, His; R, Arg; D, Asp; K, Lys; Q, Gln.bSubcellular localization of HaRxL103 alleles. GFP-tagged HaRxL103 alleles were transiently (co)expressed with/without RPP4-FLAG via agroinfiltration inN. benthamiana. Images are from GFP channel and single-plane confocal images. Scale bars, 10 μm.cHR cell death phenotypes when co-expressed of HaRxL103 alleles with RPP4 inN. benthamiana. The leaves inoculated withAgrobacteriumcontaining the indicated gene constructs were photographed under UV at 3 dpi. Protein accumulation (d), subcellular localization (e),AtPR1expression (f), andHpagrowth (g) in Arabidopsis Col-0 transgenic lines containing Est-GFP, Est-103Emoy2and estradiol-inducible GFP-HaRxL103Hind2(Est-103Hind2) constructs. Immunoblot, qRT-PCR andHpagrowth analyses were done as described in Fig.2d–f.dAsterisks indicate the detected GFP, GFP-HaRxL103Emoy2or GFP-HaRxL103Hind2constructs.eCol-0 transgenic lines pretreated with estradiol were DAPI-stained. The upper image is from the GFP channel, the middle image is from the DAPI channel, and the lower image is the overlay of the GFP and DAPI channels. Scale bars, 10 μm.fData are means ± SDs from three biological replicates. Different letters indicate significantly different values atp< 0.01 (one-way ANOVA, Tukey’s HSD).gData are means ± SEs from five biological replicates. Different letters indicate significantly different values atp< 0.01 (one-way ANOVA, Tukey’s HSD) 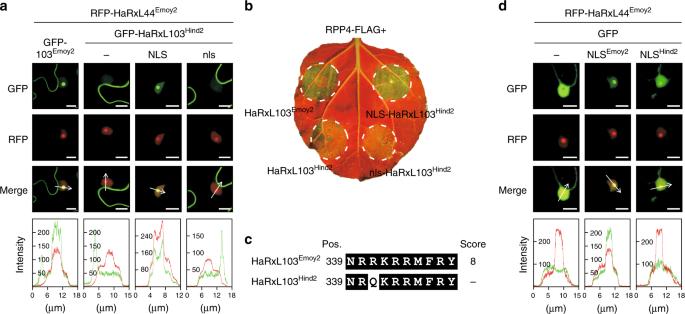Fig. 4 The mutation in HaRxL103Hind2affects in planta subcellular localization.aSubcellular localization of GFP-HaRxL103Emoy2(GFP-103Emoy2), GFP-HaRxL103Hind2, and NLS- or nls-fused GFP-HaRxL103Hind2. GFP-tagged HaRxL103Emoy2and HaRxL103Hind2variants were transiently co-expressed with RFP-HaRxL44Emoy2via agroinfiltration inN. benthamiana. The upper image is from the GFP channel, the middle image is from the RFP channel, and the lower image is the overlay of the GFP and RFP channels. Fluorescence intensity profile (GFP, green; RFP, red) across the white arrow was performed using the analyzing software (Leica, bottom). Scale bars, 10 μm.bHR cell death phenotypes when co-expressed of HaRxL103Emoy2and HaRxL103Hind2variants with RPP4 inN. benthamiana. The leaves inoculated withAgrobacteriumcontaining the indicated gene constructs were photographed under UV at 3 dpi.cA predicted NLS sequence from HaRxL103Emoy2and HaRxL103Hind2. Prediction of NLS in HaRxL103Emoy2or HaRxL103Hind2was done in cNLS Mapper. Position of predicted NLS and score for the prediction are indicated. Identical sequences are indicated in white on black.dSubcellular localization of GFP-fused predicted NLS from HaRxL103Emoy2(NLSEmoy2) and HaRxL103Hind2(NLSHind2). GFP, GFP-NLSEmoy2, and GFP-NLSHind2were transiently co-expressed with RFP-HaRxL44Emoy2via agroinfiltration inN. benthamiana. Imaging was performed as described in (a). Scale bars, 10 μm The nuclei were pelleted by centrifugation at 1500 g for 10 min at 4 °C, and the supernatant was taken as a cytoplasmic protein extract. The pellet was washed three times with nuclei wash buffer (20 mM Tris–HCl, pH 7.4, 25% glycerol, 2.5 mM MgCl 2 , 0.2% Triton X-100, 10 mM DTT, 1 mM PMSF and protease inhibitor cocktail) at 4 °C. The nuclei were then resuspended in 3 ml icecold nuclei resuspension buffer (20 mM HEPES-KOH, pH 7.9, 20% glycerol, 2.5 mM MgCl 2 , 250 mM NaCl, 0.2 mM EDTA, 0.2% Triton X-100, 10 mM DTT, 1 mM PMSF, and protease inhibitor cocktail) and then ultracentrifugated at 34,000 g for 15 min at 4 °C. The pellet was resuspended in the same buffer and subjected to sonication (parameters: output, 6; duty, 40) for 4 min. After centrifugation at 21,700 g for 30 min at 4 °C, the supernatant was taken as a nuclear protein extract. In the wash step of immunoprecipitation of cytoplasmic and nuclear protein extracts, lysis buffer and nuclei resuspension buffer were used, respectively. UGPase and Histone H3 were detected by anti-UGPase antibody (AS05 086; Agrisera) in 1:3000 dilution and anti-Histone H3 antibody (AS10 710; Agrisera) in 1:5000 dilution as markers for cytoplasmic and nuclear proteins, respectively. For the western blotting probed with antibodies against GFP and FLAG, 2 μl of cytoplasmic protein sample and 25 μl of nuclear protein sample were loaded. For the anti-UGPase and anti-Histone H3 western blotting, 5 μl of cytoplasmic protein sample and 5 μl of nuclear protein sample were loaded. Confocal microscopy For in planta subcellular localization analysis in N. benthamiana , cut leaf patches were mounted in water and analyzed on a Leica DM6000B/TCS SP5 confocal microscope (Leica Microsystems) with the following excitation wavelengths: GFP, 488 nm; RFP, 561 nm. In the case of Arabidopsis transformants containing Est-GFP, Est-103, and Est-103 Hind2 , 3-week-old transgenic lines 24 h after spray treatment with estradiol were DAPI-stained using CySain ® UV Precise P (Sysmex) by vacuum infiltration. After incubation in dark for 1 h, cut leaf patches were mounted in water and analyzed on a Leica TCS SP8 X confocal microscope (Leica Microsystems) with the following excitation wavelengths: GFP, 488 nm; DAPI, 405 nm. Creation of outcrossed progeny between Hpa Emoy2 and Cala2 For creation of outcrossed F1 progeny, mixed inoculum of Emoy2 and Cala2 was inoculated in 10-day old seedlings of an accession compatible to both Emoy2 and Cala2. Two weeks after inoculation, the leaf tissue was harvested and dried. Oospores were left to mature for 1 month before asexual progeny were recovered (the following steps). Dried leaf tissue containing the mature oospores was ground to a fine powder using a pestle and mortar. Oospore inoculum was sprinkled onto the surface of soil in pots and seeds of a susceptible genotype were sown on top. Pots were watered and stored for 2 weeks at 4 °C to break any remaining seed dormancy. Sealed trays containing the pots were incubated in a growth cabinet at 16 °C under a 10-h photoperiod. Seedlings were inspected daily for asexual conidiosporangia from 5 days post-incubation. Individual infected seedlings bearing conidiosporangiophores were harvested and the asexual inoculum was bulked on susceptible seedlings prior to testing. Putative F1 progeny were single-spored from conidiosporangia and confirmed as hybrids by a PCR-based CAPS marker using restriction enzyme BspDI and specific primers (HaRxL103_CAPS_F and HaRxL103_CAPS_R) listed in Supplementary Table 2 . 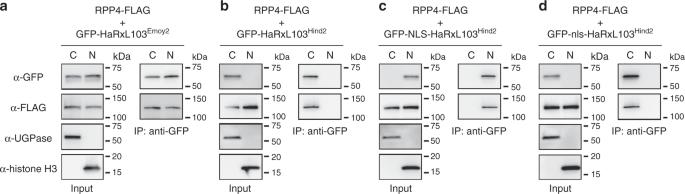Fig. 5 Interactions between HaRxL103Emoy2/HaRxL103Hind2and RPP4 in cytoplasm and/or nucleus. In planta interaction of GFP-HaRxL103Emoy2(a), GFP-HaRxL103Hind2(b), and GFP-NLS/nls-HaRxL103Hind2(c,d) with RPP4-FLAG in cytoplasm and nucleus. Cytoplasmic (C) and nuclear (N) protein extracts were separately isolated fromN. benthamianaleaves inoculated withAgrobacteriumcontaining the indicated gene constructs at 2 dpi. Co-immunoprecipitation was performed with each extract using MACS MicroBeads with GFP antibody. Anti-GFP (upper panel), anti-FLAG (the 2nd panel), anti-UGPase (the 3rd panel), and anti-Histone H3 antibodies (bottom panel) were used to detect the related proteins in the immunoprecipitates. UGPase and Histone H3 were checked as markers for cytoplasmic and nuclear proteins, respectively 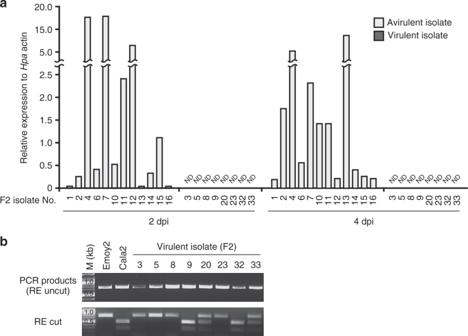Fig. 6 In an Emoy2/Cala2 F2, virulence consists with lack ofHaRxL103expression.aExpression ofHaRxL103during infection in Emoy2/Cala2 F2 individual progeny which showed virulence or avirulence on CW84:RPP4Colplants. Total RNA was prepared from the infections in Arabidopsis Ws-2eds1-1mutant at 2 or 4 dpi. qRT-PCR analysis was done as described in Fig.1c.bGenotyping of theHaRxL103locus in Emoy2/Cala2 F2 individual progeny which showed virulence on CW84:RPP4Colplants. Genotyping of theHaRxL103locus was performed by a CAPS (cleaved amplified polymorphic sequence) method. Upper and bottom panels indicate PCR products and those after restriction enzyme (RE) treatment, respectively. M marker, ND not detectable The F2 population was derived from selfing the F1 and recovering progeny as described. The F2 progeny were single-spored prior to testing on CW84 and CW84:RPP4 Col . Genotyping in F2 progeny was performed by a PCR-based CAPS marker using the same restriction enzyme and primers as above.